Stochastic switching of cantilever motion The cantilever is a prototype of a highly compliant mechanical system and has an instrumental role in nanotechnology, enabling surface microscopy, and ultrasensitive force and mass measurements. Here we report fluctuation-induced transitions between two stable states of a strongly driven microcantilever. Geometric nonlinearity gives rise to an amplitude-dependent resonance frequency and bifurcation occurs beyond a critical point. The cantilever response to a weak parametric modulation is amplified by white noise, resulting in an optimum signal-to-noise ratio at finite noise intensity. This stochastic switching suggests new detection schemes for cantilever-based instrumentation, where the detection of weak signals is mediated by the fluctuating environment. For ultrafloppy, cantilevers with nanometer-scale dimensions operating at room temperature—a new transduction paradigm emerges that is based on probability distributions and mimics nature. Noise-activated switching between two stable states in a nonlinear potential has been observed in a variety of physical systems. This process can enhance the response to weak input signals via stochastic resonance and has applications in biology, physics and information science [1] . Previously studied systems include a parametrically driven electron in a Penning trap [2] , a superconducting loop with a Josephson junction [3] and an atomic cloud in an magneto-optical trap [4] . Micromechanical doubly clamped beams and torsional resonators driven into bistability can also exhibit noise-induced switching, leading to an enhancement of the Signal-to-Noise Ratio (SNR) [5] , [6] , [8] . In torsional oscillators, the nonlinearity arises from the externally applied electrostatic driving force [6] , [7] . Recently, bistability has also been observed in microcantilevers [9] , [10] , [11] , [12] , which are omnipresent as probes in nanoscience instrumentation [13] , [14] , [15] , [16] , [17] , [18] , [19] . In a cantilever, the nonlinearity is intrinsic and originates from the cantilever geometry. A strongly driven cantilever moves in a dynamic double-well landscape [20] , where vibration states with a low- and a high amplitude are stable. We demonstrate that in this regime, the drive force fluctuations at finite temperature induce switching, which can be viewed as fluctuation-induced transitions between the attractors in the dynamic double well [7] , [20] , [21] . This opens a route towards new transduction schemes for cantilevers in the presence of noise. 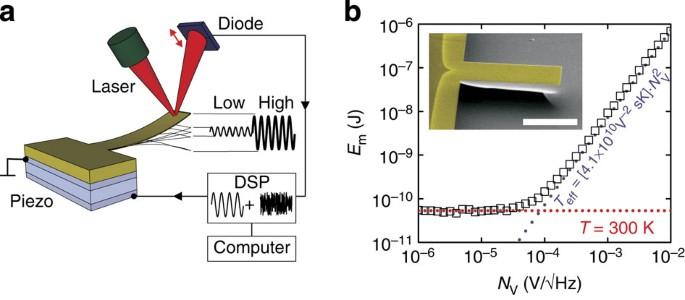Figure 1: Setup and thermometry of a noise-driven cantilever. (a) Diagram of measurement circuit. The cantilever is driven by stochastic and harmonic voltages generated in the DSP and applied to the piezoelectric crystal. Its motion is detected optically. Details on the fabrication and the setup are provided inSupplementary Fig. S1. At strong driving, two distinct states are stable, which correspond to a low and a high vibrational amplitude. (b) Inset: colourized scanning electron micrograph of a silicon nitride cantilever (scale bar 20 μm). Measured energyEm=∫ωSxx(ω′)dω′ as a function of the applied noiseNV. Whenthe energy equals the thermomechanical noise. IncreasingNVyields the quadratic dependence between effective mode temperature and the applied noise voltage according to. Figure 1a shows an example of a thin cantilever, with dimensions length × width × height ( L × w × h )=24 × 8 × 0.07 μm 3 . The device is driven by applying stochastic and harmonic voltages to a piezo actuator, at a pressure of ~10 −5 mbar. Its motion is detected by an optical deflection technique and network, and spectrum analysis of the photodiode signals is implemented in a digital signal processor (DSP). Figure 1b shows the experimental setup. The power spectral density of the cantilever displacement near the fundamental resonance frequency, f 0 =137.5 kHz, is measured when uniformly distributed white noise is applied with a spectral amplitude, N V , varying between and . The effective temperature of the fundamental mode is determined as a function of the applied noise voltage by integrating the power spectral density of the mechanical displacements (details are provided in Supplementary Fig. S1 ). For the applied noise exceeds the thermomechanical fluctuations. As expected, the energy of the mode is then proportional to the squared noise voltage; the calibrated effective temperature of the fundamental mode equals . Figure 1: Setup and thermometry of a noise-driven cantilever. ( a ) Diagram of measurement circuit. The cantilever is driven by stochastic and harmonic voltages generated in the DSP and applied to the piezoelectric crystal. Its motion is detected optically. Details on the fabrication and the setup are provided in Supplementary Fig. S1 . At strong driving, two distinct states are stable, which correspond to a low and a high vibrational amplitude. ( b ) Inset: colourized scanning electron micrograph of a silicon nitride cantilever (scale bar 20 μm). Measured energy E m =∫ ω S xx ( ω ′) dω ′ as a function of the applied noise N V . When the energy equals the thermomechanical noise. Increasing N V yields the quadratic dependence between effective mode temperature and the applied noise voltage according to . Full size image The nonlinear dynamics of the cantilever driven by a force f at frequency Ω is governed by where a is the scaled displacement, ω is the dimensionless resonance frequency ( ω =3.52) and δ the aspect ratio ( h / L ) 2 . The fourth and fifth terms represent geometric and inertial nonlinearities of the cantilever, respectively, causing the resonance frequency to increase with the vibration amplitude, as is discussed in more detail in Supplementary Fig. S1 and Supplementary Discussion 1 . As the nonlinearity is inherent in a cantilever, no externally applied nonlinear force is required, such as the weakening electrostatic force in a micromechanical torsional resonator [6] . Note that in contrast to doubly clamped beams in which the nonlinearity originates from the displacement-induced tension [5] , [22] , a cantilever is clamped on one side and therefore displaces without extending. This makes the cantilever highly susceptible to thermal fluctuations. At a critical amplitude and frequency, a cr and f cr , respectively, a bifurcation occurs [10] . Two stable states coexist beyond this point, represented by motion at a low and a high vibrational amplitude [9] , [10] , [23] . Here we show that, in this large amplitude regime, the presence of noise leads to parametric excitation, which enables transitions between the two states. A rise and decay of the switching rate is observed when the noise intensity is increased. Close to the onset of spontaneous switching, the sensitivity of the cantilever to a weak excitation is enhanced, and the SNR maximizes at finite noise intensity. Stochastic switching To study the noise-enabled transitions in the dynamic double well, we prepare the cantilever in the low state and artificially increase its temperature by applying voltage noise to the piezo (see Methods). 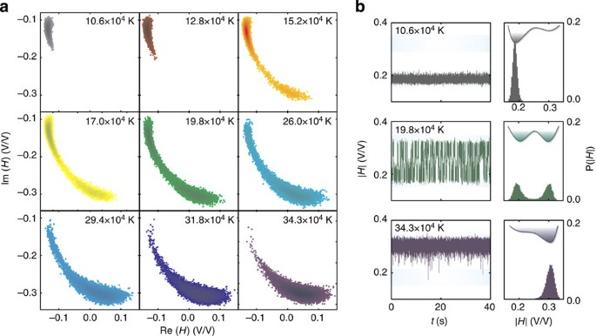Figure 2: Stochastic switching of microcantilever motion. (a) Dynamics of the noise-driven microcantilever represented in the complex plane. The cantilever moves from the low- to the high-amplitude attractor while increasing the noise power; the corresponding effective temperatures are indicated (upper left to lower right panels). Incoherent transitions occur at intermediate noise levels on the central row. (b) Time domain representation and probability densities (P) of the resonator amplitude response (|H|) for selected panels from each row. The shape of the dynamic double well is sketched in the inset. The central panel represents the symmetric system. Figure 2a shows the real and the imaginary parts of the motion for nine different noise powers, which are expressed in the effective temperature of the fundamental mode. The cantilever is driven at an amplitude a d =1.0902 a cr and a frequency f d =1.0021 f cr . For T <10.6 × 10 4 K, the cantilever resides in the low-amplitude state (upper left panel): no switching is observed within the measurement time (40s). When the noise intensity is raised, in the subsequent panels, the cantilever occasionally crosses the barrier. At T eff =19.8 × 10 4 K, the central panel, the high- and the low-amplitude states are equally probable, and switching occurs through a narrow region in the phase space [24] . The switching decays upon further increasing the noise intensity, and at T eff =43.3 × 10 4 K, the cantilever settles at the high-amplitude state. Figure 2b shows time traces (left) and histograms (right) of the amplitude response, clearly demonstrating the discrete states of low- and high-amplitude motion and the transitions between them. The responses correspond to the first, central and the last panels in Fig. 2a . Figure 2: Stochastic switching of microcantilever motion. ( a ) Dynamics of the noise-driven microcantilever represented in the complex plane. The cantilever moves from the low- to the high-amplitude attractor while increasing the noise power; the corresponding effective temperatures are indicated (upper left to lower right panels). Incoherent transitions occur at intermediate noise levels on the central row. ( b ) Time domain representation and probability densities ( P ) of the resonator amplitude response (| H |) for selected panels from each row. The shape of the dynamic double well is sketched in the inset. The central panel represents the symmetric system. Full size image The transition rates and residence times are plotted in Fig. 3 . The switching rate, shown in panel (a), rises according to Kramers law [25] upon increasing the noise intensity and maximizes at T eff =20.7 × 10 4 K to Γ max =13 s −1 , well below the relaxation rate, f 0 / Q 0 =278 s −1 , of the cantilever. In contrast to the saturation of the transition rate as is the case for a static double well [1] , [25] , a decay in the transition rate is observed upon increasing the noise level, which indicates that the noise is no longer purely additive but gains a multiplicative character at high intensities. 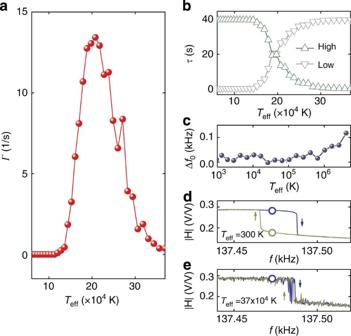Figure 3: Transition rates and residence times. (a) Transition rate,Γ, as a function of temperature, computed for 20,000 samples. (b) Residence time,τ, in the states of high-amplitude- and low-amplitude motions. (c) Resonance frequency of the noise-driven cantilever as a function of the effective temperature. (d,e) Bistable frequency response lines of the cantilever measured at room temperature (d)Teff=37 × 104K (e). Increasing the temperature affects the double well: the initially bistable system, marked by the circle, is monostable at a high noise intensity. Figure 3: Transition rates and residence times. ( a ) Transition rate, Γ , as a function of temperature, computed for 20,000 samples. ( b ) Residence time, τ , in the states of high-amplitude- and low-amplitude motions. ( c ) Resonance frequency of the noise-driven cantilever as a function of the effective temperature. ( d , e ) Bistable frequency response lines of the cantilever measured at room temperature ( d ) T eff =37 × 10 4 K ( e ). Increasing the temperature affects the double well: the initially bistable system, marked by the circle, is monostable at a high noise intensity. Full size image Quenching of the hysteresis To investigate the origin of the switching rate decay, we start with a measurement of the resonance frequency of the noise-driven cantilever as a function of the noise intensity, without applying the periodic driving force. Figure 3c , shows the result: starting at T eff ≈20 × 10 4 K, the excessive noise causes an upward shift in the resonance frequency, resulting from nonlinearity. To investigate whether this frequency shift affects the dynamic double well, we measure the cantilever response to forward and backward frequency sweeps, at low and high noise intensities. Comparing the responses, shown in Fig. 3d,e , following two effects are visible: the noise reduces the hysteresis, as is expected for a double-well energy potential and as observed in dynamically bistable doubly clamped beams [26] . In addition, the hysteretic regime shifts to a higher frequency and amplitude, and this causes an increase in the critical driving force a cr . Thus, a system prepared in a dynamic double well in the presence of weak fluctuations, as indicated by a white dot in the upper panel, becomes monostable when the noise intensity is increased. A detailed measurement of the hysteretic regime at different noise intensities, presented in Fig. 4 , confirms this mechanism. Frequency stiffening becomes significant around T eff =20 × 10 4 K, close to where the peak in the switching rate is observed. A decay in switching rate in the limit of high noise powers was also observed in magnetomotive-driven doubly clamped nanomechanical resonators [5] , and here we demonstrate that such effects are expected as excitation by excessive noise affects the effective spring constant. 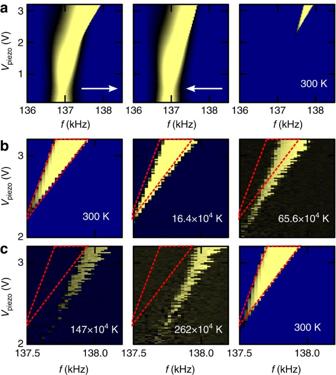Figure 4: Quenching of the hysteretic regime. (a) Cantilever susceptibility (response magnitude normalized to the drive force) at room temperature. The frequency is swept along the horizontal (fast) axis, whereas after each trace, the drive strength is incremented (vertical, slow axis). Arrows indicate the sweep direction. The third panel shows the hysteretic regime by superimposing the data of forward and backward sweeps. Bifurcation occurs atacr=2.115 V andfcr=137.31 kHz. (b) Hysteretic regime at indicated effective temperatures, starting and ending with a measurement at room temperature (300 K). Figure 4: Quenching of the hysteretic regime. ( a ) Cantilever susceptibility (response magnitude normalized to the drive force) at room temperature. The frequency is swept along the horizontal (fast) axis, whereas after each trace, the drive strength is incremented (vertical, slow axis). Arrows indicate the sweep direction. The third panel shows the hysteretic regime by superimposing the data of forward and backward sweeps. Bifurcation occurs at a cr =2.115 V and f cr =137.31 kHz. ( b ) Hysteretic regime at indicated effective temperatures, starting and ending with a measurement at room temperature (300 K). 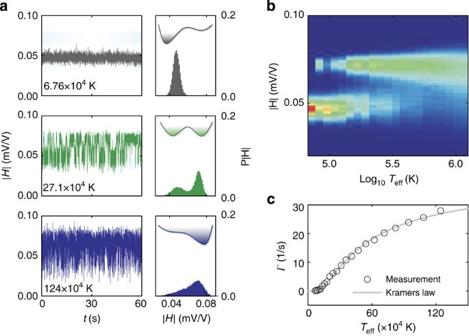Figure 5: Experiments with a different device. (a) Stochastic switching of a cantilever with dimensionsL×w×h=26 × 8 × 0.07 μm3, withf0=143.6 kHz,Q0=1,537 and an effective temperature. The probability density and the switching rate are computed from 20,000 samples. ForTeff<105K, the cantilever vibrates in the low-amplitude state and no switching is observed within the time of the experiment (180 s). AtTeff=27.1 × 104K, the cantilever states are equally populated, and when the noise level is further increased, the high state becomes more probable. (b) Histograms for a range of noise intensities; colourscale: P(|H|). (c) Kramers law fits to the switching rate. Full size image Figure 5 shows measurements on a second device, driven stronger at a =1.34 a cr and f =1.00016 f cr . Here the fluctuations are strong enough to access the unstable state, and the switching rate continues to follow Kramers law [25] over a longer range of noise intensities. This behaviour is predicted for a dynamic double well [20] and was observed in doubly clamped nanomechanical resonators and parametric oscillators [24] , [26] . In the limit of low noise, Kramers law effectively describes the stochastic switching, and the switching rate is given by Γ = Γ 0 , with Γ 0 =39 s −1 and T 0 =4.6 × 10 5 K. In this experiment, the switching rate becomes comparable to the relaxation rate of the cantilever, f 0 / Q 0 =93 s −1 . These experiments indicate that in the dynamic double well, the stochastic switching between stable states occurs in a limited regime of noise powers. Figure 5: Experiments with a different device. ( a ) Stochastic switching of a cantilever with dimensions L × w × h =26 × 8 × 0.07 μm 3 , with f 0 =143.6 kHz, Q 0 =1,537 and an effective temperature . The probability density and the switching rate are computed from 20,000 samples. For T eff <10 5 K, the cantilever vibrates in the low-amplitude state and no switching is observed within the time of the experiment (180 s). At T eff =27.1 × 10 4 K, the cantilever states are equally populated, and when the noise level is further increased, the high state becomes more probable. ( b ) Histograms for a range of noise intensities; colourscale: P(| H |). ( c ) Kramers law fits to the switching rate. Full size image Noise-enabled measurements Noise-enabled measurements, similar to the ones demonstrated in doubly clamped beams [5] , [26] , [27] , [28] , are now implemented in cantilevers. The sensitivity of these instruments is ultimately limited by the thermomechanical fluctuations of the cantilever, and here we demonstrate a scheme that exploits such fluctuations. To demonstrate noise-enabled detection in a cantilever, the cantilever is prepared in a bistable state by driving it at a d =1.0596 a cr and f d =1.0022 f cr . The double well is then parametrically perturbed by a weak and slow sinusoidal amplitude modulation (amplitude 5 mV, period 6 s) of the periodic excitation signal on the piezo. This perturbation mimics, for instance, a small force to be detected by the cantilever-based instrument. 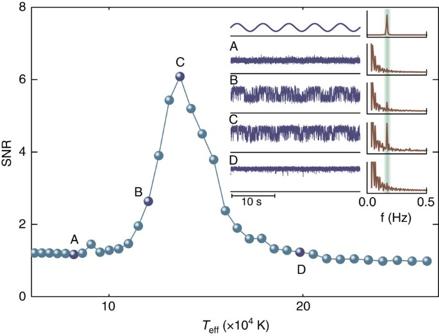Figure 6: Noise-enhanced measurement of subthreshold cantilever excitations. Inset: top row shows the excitation signal in time (left) and frequency (right) domains. The cantilever response at increasing noise intensity is shown in panels (A–D). Main figure: SNR as a function of the effective temperature. Figure 6 (inset) shows the excitation voltage in the time and frequency domains (upper panels). Panels A–D show the response for four different noise intensities close to the regime where spontaneous switching occurs; the noise intensity increases from panel A to panel D. In panel A, the cantilever vibrates in the low state: the modulation of the double well is too weak to cross the barrier and only an incidental escape to the high-amplitude state is observed. In panel B, occasional transitions occur, weakly locked to the modulation signal. In C, the transitions are synchronized to the modulation. Here the amplification of the cantilever response by the noise is maximized. Further increasing the temperature shifts the double well and directs the cantilever to the high state (D). A fast Fourier transform of the detected signals ( Fig. 6 (inset), right column) clearly reveals the synchronization observed in panel C: the cantilever response peaks at the excitation frequency. The SNR is calculated as ref. 1 Figure 6: Noise-enhanced measurement of subthreshold cantilever excitations. Inset: top row shows the excitation signal in time (left) and frequency (right) domains. The cantilever response at increasing noise intensity is shown in panels (A–D). Main figure: SNR as a function of the effective temperature. Full size image where is the height of the power spectrum peak at the modulation frequency , and is the spectral background. Figure 6b shows the SNR as a function of the temperature. A peak is observed at an effective temperature 13.7 × 10 4 K, in which the random fluctuations induce coherence between the cantilever motion and the subthreshold excitation. In this experiment, the SNR improves by a factor of 6 at the optimum noise level. The experiments described in this work are carried out at elevated temperatures, obtained by artificially heating the mechanical system. In contrast to doubly clamped structures such as silicon nitride strings, the amplitude of a cantilever is not restricted by the displacement-induced tension, and this makes large thermomechanical amplitudes possible. The limited dynamic range of NEMS resonators is a recognized disadvantage, and methods to enhance it are actively studied [9] , [22] , [29] , [30] . When the fluctuations are strong enough to quench the regime of linear motion, the dynamic range of the cantilever approaches zero. A critical temperature can be defined for which the amplitude of the thermal fluctuations approaches the critical amplitude for bistability. The critical amplitude for a cantilever [9] equals , and this value should thus be compared with the amplitude of the thermomechanical fluctuations, . One then finds that the crossover temperature scales with the cantilever dimensions as , assuming a constant Q . Scaling the thickness h , of the present devices down by a factor of 100, the dynamic range is zero at room temperature. Few-layer graphene may be a viable route towards devices operating in this regime. New transduction principles are then required, which involve probabilities and switching rates rather than the deterministic input–output relations of linear and weakly nonlinear transducers. The present work demonstrates some of the characteristic aspects of this new class of mechanical systems. Cantilever fabrication and motion detection Thin cantilevers with a rectangular cross-section are fabricated by standard nanofabrication techniques, comprising low-pressure chemical vapour deposition of silicon nitride, patterning by electron beam lithography and reactive ion etching. The cantilevers are released from the silicon substrate by wet-etching the silicon in a potassium hydroxide solution (main device) or by under-etching the silicon substrate in an SF 6 /O 2 inductively coupled plasma (device of Fig. 5 ). The cantilever motion is detected using an optical deflection technique, comprising a diode laser ( λ =658 nm), an optical isolator, a polarizing beam splitter and a quarter wave plate. The laser is focused on the cantilever using a microscope objective (NA=0.6, 50 × , focal distance 11 mm). The cantilever is placed on top of a piezoelectric crystal in a vacuum chamber with a transparent window. The reflection from the cantilever is collimated by the same objective lens, passes through the wave plate and reflects from the beam splitter on a two-segment photodiode. Excitation and detection of motion The noise and the driving signals are generated separately using two DSPs. The noise is uniformly distributed and white within a bandwidth of 0–1,000 kHz. The noise spectral density and the probability density were confirmed by frequency and time domain measurements of the DSP output signal. To avoid the excitation of higher vibration modes of the cantilever, the signal is low-pass filtered at 400 kHz using four-pole Butterworth filter. The mechanical motion of the cantilever is expressed as a complex susceptibility H , which is defined as the detected photodiode signal in volts, normalized to the driving voltage applied to the piezo. A map is created of the hysteretic regime, as is shown in Fig. 4 , and subsequently the parameters of the periodic driving signal, a d and f d , are chosen within the hysteretic regime and close to the kinetic phase transition point, where the states are equally occupied [20] . The measurements of Fig. 2 , panels a and b, are taken at the same initial conditions, in which the low state is initially stable. Turning on and off the driving signal did not alter the behaviour. Changing the initial conditions—that is, the driving amplitude and frequency—results in no switching or in switching commencing at a lower or a higher effective noise temperature. Such a behaviour is expected, as the activation barrier scales exponentially with the detuning from the critical point. The robustness of the observed behaviour was verified by measuring three-dimensional histograms, similar to the one presented in Fig. 5b , for several devices. How to cite this article: Venstra, W. J. et al. Stochastic switching of cantilever motion. Nat. Commun. 4:2624 doi: 10.1038/ncomms3624 (2013).